Another rapid event in the carbon-14 content of tree rings Previously, we have observed that the atmospheric 14 C content measured in tree rings showed a strong increase from AD 774 to 775. Although the cause of this event can be explained by a large solar proton event or a short gamma-ray burst, a more detailed discussion of the cause is difficult because the rate of occurrence of such rapid 14 C events remains unknown. Here we report new 14 C measurements from AD 822 to 1021, and the discovery of a second rapid increase of 14 C content from AD 993 to 994. The 10 Be flux in the Antarctic ice core shows peaks corresponding to these two 14 C events. The proportions of flux increase ( 14 C/ 10 Be) of the two events are consistent with each other. Therefore, it is highly possible that these events have the same origin. Considering the occurrence rate of 14 C increase events, solar activity is a plausible cause of the 14 C increase events. Radiocarbon 14 C is produced in the Earth’s atmosphere by nuclear interactions with galactic cosmic rays, most of which are charged particles. The flux of cosmic rays is modulated by the solar magnetic activity and the geomagnetic field. Radiocarbon oxidizes in the atmosphere to form 14 CO 2 and is taken up by trees as a part of the global carbon cycle. As 14 C is a radioisotope with a half-life of 5,730 years, the 14 C content in tree rings provides a record of cosmic ray intensity and solar activity over a few tens of millennia. While the solar magnetic activity and the geomagnetic field modulate the cosmic ray background, high-energy phenomena, such as gamma-ray events and large solar proton events (SPEs), can produce a large number of cosmic rays all at once. Then, if such events have occurred in the past, the 14 C content in tree rings is possible to record the rapid increase due to the events. Recently, we found a rapid increase in 14 C content within 1 year from AD 774 to 775 (ref. 1 ). The possible cause of the event is a supernova or a large SPE. However, neither a local supernova nor a large SPE is likely responsible, because of a lack of record of corresponding supernova or supernova remnant and too high energy for SPE [1] (ref. 1 ). There have been some attempts to specify the cause of the AD 775 event. Melott and Thomas [2] have reexamined the flare energy of the AD 775 event by assuming a directional flare with opening angle of 24°, and concluded that implied energy of SPE is reduced to ~10 33 erg. This is about 1/100 energy of our calculation [1] , which presumes that flare particles propagated isotropically. Then SPE appears to be the possible cause of the AD 775 event [2] . Some studies also show the SPE origin [3] , [4] . On the other hand, although we considered only the normal supernova origin [1] , Hambaryan and Neuhauser [5] claim that a short gamma-ray burst (GRB) (<2 s) can explain the AD 775 event. Although the cause of this event can be explained by a large SPE [2] , [3] , [4] or a short GRB [5] , a more detailed discussion of the cause is difficult because the rate of occurrence of such rapid 14 C events remains unknown. We need to know whether more events similar to the AD 775 event exist in the past 14 C record. Although the 14 C increment around AD 775 is the largest class in the last three millennia from IntCal09 data (which is a data set back to about 25,000 years BP) [6] , there are a large number of period when the 14 C content has not been measured with 1-year resolution. Therefore, it is possible that smaller increases than the AD 775 event are hidden in these unmeasured periods. These small increases will not be detected until after 1-year resolution measurements. Here, we report the measurement of 14 C content during an extended period from AD 822 to 1021 to search other 14 C increase events, and found another rapid increase from AD 993 to 994. Considering the occurrence rate of the 14 C increase events, the large SPE is a plausible cause of the 14 C events. Measurement data We collected a new series of biennial measurements of 14 C content in the Japanese cedar tree ( Cryptomeria japonica ), which is the same tree as that used for the AD 775 event [1] , from AD 822 to 1021. In addition to these measurements, we also measured annual resolution data from AD 991 to 1001 in the same tree. The information about the sample is shown in Supplementary Table S1 and Supplementary Fig. S1 . As the 14 C data for AD 600 to 820 have been already measured [1] (Miyake, F., Masuda, K. and Nakamura, T. manuscript in preparation), we obtained a continuous series of AD 600 to 1021. We have updated our previous series [1] by measuring new data (for even years: AD 752–768, 782–788 and 794–820, and for odd years: AD 767 and 769). As data for AD 896 and 898 do not exist, we obtained values of 14 C content (which is described as Δ 14 C (refs. 7 ) for those years by a linear interpolation method. As the data for overlapping years match within measurement errors, these series of measurements are reproducible and we applied weighted averaging for the same year. 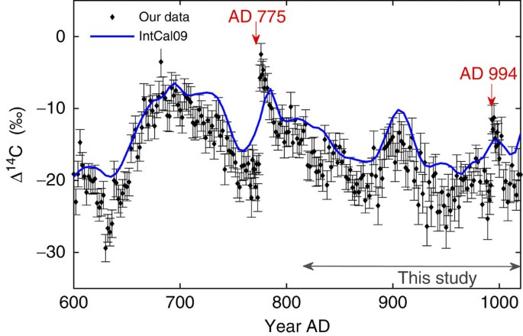Figure 1:14C data from AD 600 to 1021. Diamonds show our results, which are obtained by a weighted mean of the 2–5 series. The blue curve represents the IntCal09 data set6. The errors are the resultant of error propagation. The error for a sample is a statistical error from a Poisson distribution, and the error for the standard sample is the greater one of either averaged statistical error from Poisson distribution of Δ14C for the six standard samples or the s.d. of values of14C/12C for six standard samples. Figure 1 shows the consolidated Δ 14 C data of some series for the period of AD 600 to 1021. Figure 1: 14 C data from AD 600 to 1021. Diamonds show our results, which are obtained by a weighted mean of the 2–5 series. The blue curve represents the IntCal09 data set [6] . The errors are the resultant of error propagation. The error for a sample is a statistical error from a Poisson distribution, and the error for the standard sample is the greater one of either averaged statistical error from Poisson distribution of Δ 14 C for the six standard samples or the s.d. of values of 14 C/ 12 C for six standard samples. Full size image The first half of Fig. 1 shows a grand solar minimum from AD 650 to 720 (Miyake, F., Masuda, K. and Nakamura, T. manuscript in preparation) and a rapid increase of 14 C content from AD 774 to 775 (refs. 1 ). The second half of Fig. 1 shows a rapid increase of 9.1% in 14 C content from AD 993 to 994. This is a clear increase that is outside the measurement error (5.1 σ ). A comparison of the AD 775 and the AD 994 events is shown in Supplementary Table S2 and Fig. 2 . The shapes of the two series are very similar, that is, a rapid increase within 1 year followed by a decay owing to the carbon cycle. The scale of the AD 994 event is 0.6 times as large as the AD 775 event. 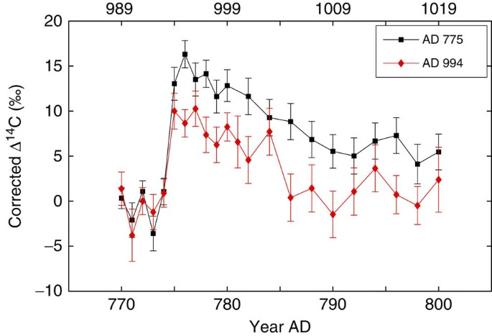Figure 2: Comparison of the AD 775 and the AD 994 peaks. Squares show the AD 775 series from AD 770–800, and diamonds show the AD 994 series from AD 989–1019. The zero level of the vertical axes is shifted to be the weighted mean value of AD 770–774 for the AD 775 series and AD 989–993 for the AD 994 series. The errors are the resultant of error propagation. The error for a sample is a statistical error from a Poisson distribution, and the error for the standard sample is the greater one of either averaged statistical error from Poisson distribution of Δ14C for the six standard samples or the s.d. of values of14C/12C for six standard samples. Figure 2: Comparison of the AD 775 and the AD 994 peaks. Squares show the AD 775 series from AD 770–800, and diamonds show the AD 994 series from AD 989–1019. The zero level of the vertical axes is shifted to be the weighted mean value of AD 770–774 for the AD 775 series and AD 989–993 for the AD 994 series. The errors are the resultant of error propagation. The error for a sample is a statistical error from a Poisson distribution, and the error for the standard sample is the greater one of either averaged statistical error from Poisson distribution of Δ 14 C for the six standard samples or the s.d. of values of 14 C/ 12 C for six standard samples. Full size image Comparison with IntCal data set Although the quasi-decadal IntCal09 data set [6] shows a small 14 C enhancement around AD 994 (3 permil increase from AD 980 to 995), this increase is hardly distinguishable from many other variations. To compare our results (obtained from Japanese trees) with IntCal98 (obtained from North American and European trees) [8] , we averaged the yearly data to obtain a series with a decadal time resolution. The result from AD 605 to 1015 is shown in Fig. 3 . The two series show similar variations to each other; however, our results are 2.1 permil smaller than IntCal98 on average (this is 7.0 σ significance level). This is considered as a regional effect. As Yaku-Island, where our sample trees lived, is located in southern Japan and is surrounded by ocean, its atmosphere is affected by marine low 14 C level gas [9] . 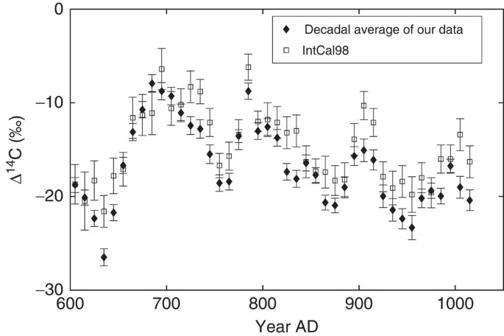Figure 3: Comparison of our result with IntCal98 data. The vertical axis represents the14C content (in Δ14C), and the horizontal axis represents the calendar year. Open squares show the IntCal98 data and filled diamonds show the decadal average of our data (AD 600–1021). Figure 3: Comparison of our result with IntCal98 data. The vertical axis represents the 14 C content (in Δ 14 C), and the horizontal axis represents the calendar year. Open squares show the IntCal98 data and filled diamonds show the decadal average of our data (AD 600–1021). Full size image The 14 C content measurements for the recorded ages of supernova explosions (SN1006, SN1054, SN1572, SN1604 and SN1885) (refs. 10 , 11 12 ) and the emergence years of large solar flares (the Carrington flare (SPE1859) that occurred in AD 1859, and SPE1460 that was detected by annual 10 Be data [3] , [13] , [14] ) (refs. 12 , 15 , 16 ) have been conducted (as shown in Supplementary Fig. S2 ). We also measured the 14 C content around SN1054 and SPE1859 using another Japanese cedar tree (Tree-C, information of this sample is shown in Supplementary Table S1 ). However, none of the 14 C contents show rapid increases within 1 year. There is no 14 C increase within 1 year during other periods, from AD 1374 to 1954 (refs. 12 , 15 , 16 , 17 ). Only rapid 14 C increases within 1 year in AD 775 and 994 have been found during about 1,600 years (when we have 1- or 2-year resolution 14 C data). Another cosmogenic nuclide, 10 Be, in the Antarctic Dome Fuji ice core also shows increases in the flux corresponding to around AD 775 and AD 994 (refs. 18 ). 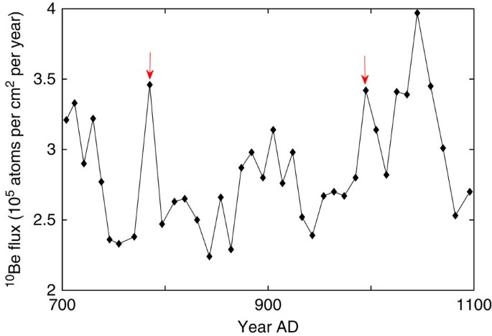Figure 4:10Be data from ice core of Dome Fuji in Antarctica. The vertical axis represents the10Be flux, which is calculated from the snow accumuration rate, estimated by the three-point (1.5 m: ~;30 years) averaged δ18O (refs.5). The horizontal axis represents the calendar year. Each point is corrected by a10Be–14C correlation age model. The two arrows show the ages of AD 785 and AD 995. The10Be flux increments of the two data is 1.08 × 105(atoms per cm2per year) from AD 770 to 785 and is 0.72 × 105(atoms per cm2per year) from AD 985 to 995. Figure 4 shows 10 Be flux data for AD 700–1100. The ages of the 10 Be data are determined by matching the production rate pattern of 10 Be with the 14 C production [18] . The increasing rates are 7.2 × 10 3 (atoms per cm 2 per year/year) from AD 770 to 785, and 6.2 × 10 3 (atoms per cm 2 per year/year] from AD 985 to 995. The scale of the increase around AD 994 is 0.86 times as large as that around AD 775. This value is consistent with the ratio for 14 C events (0.6 times larger) because 10 Be data have a lower time resolution (~;10 years resolution) than that of 14 C data. If the causes of two events are different, the difference between the ratios of 14 C and 10 Be production rates is expected. This difference is occurred by energy spectrums or particle species of the origin events. From the consistency of increasing ratio of AD 775 and 994 between 14 C and 10 Be, the cause of the two events must be same. Figure 4: 10 Be data from ice core of Dome Fuji in Antarctica . The vertical axis represents the 10 Be flux, which is calculated from the snow accumuration rate, estimated by the three-point (1.5 m: ~;30 years) averaged δ 18 O (refs. 5 ). The horizontal axis represents the calendar year. Each point is corrected by a 10 Be– 14 C correlation age model. The two arrows show the ages of AD 785 and AD 995. The 10 Be flux increments of the two data is 1.08 × 10 5 (atoms per cm 2 per year) from AD 770 to 785 and is 0.72 × 10 5 (atoms per cm 2 per year) from AD 985 to 995. Full size image Possible causes of these 14 C events are large SPEs or cosmic gamma-ray events [1] . For gamma-ray events, there are supernova explosions and GRBs [5] . The supernova remnants corresponding to AD 775 and 994 have not been detected ( http://hea-www.harvard.edu/ChandraSNR/snrcat_gal.html (Chandra Supernova Remnant Catalog)) [19] and historical documentation has not been found [20] . Therefore, a supernova origin is quite unlikely [1] , [5] . Although only the normal supernova origin was considered in Miyake et al . [1] , Hambaryan and Neuhauser claim that a short GRB (<2 s) can explain the AD 775 event [5] . In case of a short GRB, its spectral hardness is consistent with the differential production rates of 14 C and 10 Be, and the absence of historical records of a supernova or a supernova remnant is consistent with a short GRB [5] . Although they claim that the observed rate of short GRBs (one event in 3.75 × 10 6 years [5] ) and that of 14 C events (one 14 C event in 3,000 years) are consistent within 2.6 σ (refs. 4 ), the finding of the second 14 C event makes a 14 C event rate large, and the consistency between the observed rate of short GRBs and the 14 C event rate becomes worse (the probability of a short GRB rate with one 14 C event in 1,500 years is 0.04%). Adding to this, it is possible that the 14 C event rate is larger because there are many periods without a 1-year resolution measurement of 14 C content in the 3,000-year period. The actual 14 C event rate should be 1/800 years (detected event/measured period with 1–2-year resolution), and the probability is 0.02%. Melott and Thomas [2] also discuss the event rate of short GRB (a probablility of order 10 −4 over 1,250 years); however, their rate is lower than Hambaryan and Neuhauser. Then, the short GRB is less likely to be the cause. In addition, Hambaryan and Neuhauser claim that it is possible that more short GRBs exist than those observed, which would explain the inconsistency in the event rate between the observed short GRB rate and the 14 C event rate; however, additional studies are necessary to confirm this claim. Next, we consider the SPE origin. An emergence of SPE is considered to be closely bound to solar activity, such as solar flares and CMEs. To know the solar activity during 8–10th centuries, we have examined the IntCal data set [6] . The variation of 14 C content (which is closely related to the flux of galactic cosmic rays reaching the earth) is mainly modulated by the solar magnetic activity and the geomagnetic field. The 14 C variation in the past several hundred years reflects the solar magnetic activity as indicated by the sunspot records. In particular, periods of solar inactivity known as grand solar minima can be identified as large peaks in the past 14 C content record. The period from the late 13th century to the early 19th century is known as ‘little ice age’, which includes the Wolf, Spörer, Maunder and Dalton solar minima. On the other hand, the 8–10th centuries have no grand solar minimum. There have been some attempts to reconstruct the solar activity by using 14 C data set [21] , [22] , and they showed higher solar activity levels during the 8–10th centuries than that during the 13–19th centuries, on average. This fact may explain why the 8–10th centuries have two rapid increases of 14 C content and after the 11th century there were no such events. Based on a reassessment of an energy spectrum of SPE, production calculations of 14 C and 10 Be, and a deposition model, Usoskin and Kovaltsov [3] claimed that the AD 775 event can be explained by an extreme SPE that was about 50 times larger than the largest SPE in AD 1956. From this aspect, the AD 994 event is about 30 times larger than SPE 1956. The energetic level does not have a serious effect on living matter on the earth [2] . Also, according to Usoskin and Kovaltsov [3] , the occurrence rate of the SPE775 event is 10 −4 per year and that of the SPE994 event is 10 −3 per years. It is possible that these events occur within 200 years assuming that SPEs are mutually independent. Although they claimed that there is no apparent relationship between the occurrence of SPE and the solar activity level, or it is proposed that large SPEs are occurred more likely during grand solar minima [23] , [24] , [25] , we doubt these claims because the two events occurred in the non-solar minimum period. Considering the 14 C event rate and higher solar activity in the 8–10th centuries, a solar origin is a plausible cause of 14 C increase events. Detection of the second 14 C event indicates the possibility that a lot of smaller 14 C increases are hidden in the periods when the 14 C content has not been measured with a 1-year resolution. In the future, it will be necessary to conduct investigations of 14 C records during additional unmeasured periods with a 1-year resolution. Sample preparation To measure 14 C content in tree rings, we have to extract graphite from the wood samples. First, we separated each annual ring using a cutter knife. Then, we obtained cellulose, which does not move between rings after the rings are formed, by applying a chemical wash for each wood slice. The chemical wash consists of ultrasonic cleaning, acid–alkali–acid treatments, sodium chlorite treatment and neutralization process. The treated material was combusted to CO 2 and purified in vacuum lines. Finally, purified CO 2 is graphitized by hydrogen reduction under the catalytic influence of iron powder. AMS measurement We measured the 14 C content in extracted graphite using an accelerator mass spectrometer (AMS) at the Center for Chronological Research [26] . As AMS provides a relative measurement, six standard samples (NIST SRM4990C oxalic acid, the new NBS standard) were measured in the same batch. Two blank samples were also measured to determine the background (commercial oxalic acid was obtained from Wako Pure Chemical Industries). The concentration of 14 C expressed as Δ 14 C, which is the age- and isotopic fractionation-corrected value, was calculated according to the method by Stuiver and Polach [7] . The typical precision of 14 C content measurements was 2.8‰. How to cite this article: Miyake, F. et al . Another rapid event in the carbon-14 content of tree rings. Nat. Commun. 4:1748 doi: 10.1038/ncomms2783 (2013).